Innate immunodeficiency following genetic ablation ofMcl1in natural killer cells The cytokine IL-15 is required for natural killer (NK) cell homeostasis; however, the intrinsic mechanism governing this requirement remains unexplored. Here we identify the absolute requirement for myeloid cell leukaemia sequence-1 ( Mcl1 ) in the sustained survival of NK cells in vivo . Mcl1 is highly expressed in NK cells and regulated by IL-15 in a dose-dependent manner via STAT5 phosphorylation and subsequent binding to the 3′-UTR of Mcl1 . Specific deletion of Mcl1 in NK cells results in the absolute loss of NK cells from all tissues owing to a failure to antagonize pro-apoptotic proteins in the outer mitochondrial membrane. This NK lymphopenia results in mice succumbing to multiorgan melanoma metastases, being permissive to allogeneic transplantation and being resistant to toxic shock following polymicrobial sepsis challenge. These results clearly demonstrate a non-redundant pathway linking IL-15 to Mcl1 in the maintenance of NK cells and innate immune responses in vivo . Innate immune cells are responsible for pathogen detection, rapid inflammation and priming of sterilizing immunity in vertebrates. Innate lymphoid cells (ILCs) represent a diverse family of bone marrow-derived lymphocytes whose development depends on expression of the inhibitor of DNA-binding 2 (Id2) and cytokine signalling via the gamma common (γC) receptor [1] . ILCs are grouped into three subsets (ILC1–3) based on their functions and dependency on specific transcription factors [2] . ILCs do not express antigen receptors that are formed from rearrangement of gene segments and, thus, rely primarily on cytokines, not antigenic stimulation, to dictate their development, activation and homeostasis. Natural killer (NK) cells are the most prevalent ILC member (ILC1) being capable of spontaneous cytokine, chemokine and lytic granule production upon activation [3] . NK cell development takes place in the bone marrow of adults and requires the pleiotropic cytokine, interleukin-15 (IL-15) [4] , [5] with high expression of the IL-15Rβ chain (CD122), an essential component of IL-15 signalling [6] induced soon after commitment to the NK cell lineage [7] . IL-15-responsive progenitors need to express dimers of IL-2Rβ and the common gamma chain (γ c /IL-2Rγ/CD132) and receptor proximal kinases (Jak1/3) and Signal Transducer and Activator of Transcription 5 (STAT5A/B) in order to survive, expand and differentiate [8] . Deletion of IL-15 or IL-15Rα in vivo largely blocks NK cell development in mice; however, when IL-15 −/− or IL-15Rα −/− progenitors were transferred into wild-type mice, NK cell development was partially restored indicating a role for IL-15 and IL-15Rα ‘in trans’ expressed by non-haematopoietic cells [9] , [10] , [11] , [12] , [13] . Both IL-2 and IL-15 utilize IL-2Rγ/β heterodimers to transmit proliferative and survival signals to NK cells and have been shown to induce, enhance or maintain various members of the Bcl-2 family of anti-apoptotic proteins including Bcl-2, Bcl-xL and Mcl-1 (refs 14 , 15 , 16 , 17 , 18 , 19 , 20 ). On the flipside, we previously proposed that IL-15 regulates NK cell survival by inhibiting the activation of the BH3-only protein Bim [14] . In this instance, Bim protein levels dramatically increased in NK cells upon removal of IL-15 correlating with accelerated apoptosis. Stimulation of NK cells with IL-15 induced activation of the PI3K and MAPK pathways with phospho-Erk1/2 being responsible for Bim phosphorylation and degradation, whereas IL-15 mediated activation of the PI3K pathway was required to phosphorylate and inhibit Foxo3a (also called FKHR-L1), a member of the family of Forkhead box class O transcription factors known to induce Bim (Bcl2l11) transcription [21] . The dependency on Bim for NK cell apoptosis is evident by the resistance of Bim −/− NK cells to cell death in the absence of IL-15 and their ability to persist when transferred in IL15 −/− mice [14] . IL-7, IL-15 and IL-2 are known to promote the survival of various T-cell subsets with upregulation of Mcl-1 observed following stimulation with these cytokines and deletion of Mcl1 in differentiated T cells resulting in a significant reduction in their numbers in vivo [22] , [23] , indicating a key requirement for Mcl-1 in their steady-state survival. In addition to the well-characterized outer mitochondrial membrane role of Mcl-1 in antagonizing apoptotic proteins such as Bak, Bim and Noxa, it was recently proposed that the inner amino-terminally truncated isoform of Mcl-1 is imported into the mitochondrial matrix where it participates in mitochondrial fusion, ATP production and respiration [24] . We hypothesized that IL-15-mediated signalling is essential for NK cell homeostasis in vivo by primarily regulating the level of the highly labile anti-apoptotic protein Mcl-1 in vivo . Using a novel Mcl1-hCD4 mouse strain, whereby Cre-mediated deletion of the Mcl1 -coding sequence results in surface expression of human CD4 (hCD4) under control of the Mcl1 regulatory elements [25] , [26] , we conclusively demonstrate that Mcl1 expression is directly regulated by IL-15 via STAT5 binding to its 3′ untranslated region (UTR). The in vivo consequence of failing to express Mcl1 in differentiated NK cells was explored using Ncr1 (NKp46)-mediated deletion ( Ncr1-Cre ) of Mcl1 . NK cells are completely absent from all tissues when both copies of Mcl1 are deleted. This result in itself represents a milestone for the NK cell field, as this is the first genetic model specifically and constantly lacking NK cells. Our findings underline the non-redundant role for Mcl1 in NK cell survival downstream of IL-2Rγ/β and permit the accurate investigation into the in vivo role of NK cells during pathogenesis. NK cells express high Mcl1 levels throughout development To investigate cytokine-mediated survival in ILCs in vivo , we focused on NK cells since their development is dependent on a single growth factor (IL-15), their differentiation is well characterized and they are abundant in lymphoid organs of mice [3] . Peripheral NK cell maturation is defined by differential expression of Mac-1, CD27 and KLRG1 with immature (Imm.) NK cells being Mac-1 − CD27 + KLRG1 − , Mature 1 (M1) NK cells being Mac-1 + CD27 + KLRG1 − and Mature 2 (M2) being Mac-1 + CD27 − KLRG1 + ( Fig. 1a ) [27] , [28] , [29] . Measurement of mRNA levels of Bcl-2 family members revealed that Mcl1 is highly expressed in NK cells, and that this expression increases with maturation ( Fig. 1b and Supplementary Fig. 1 ). To visualize Mcl1 expression in vivo , we utilized a Mcl1-floxed-hCD4 mouse strain (allele is termed Mcl1 fl from herein). In this system, Cre-mediated deletion of the Mcl1 -coding sequence results in surface expression of hCD4 (hCD4) under control of the Mcl1 regulatory elements [25] , [26] . This strain was bred to the Rosa26 Cre-ERT2 ( CreERT2 ) mice to facilitate Mcl1 deletion in vivo . Treatment of Mcl1 fl/+ CreERT2 mice with tamoxifen via oral gavage resulted in stable expression of hCD4 (reporting on Mcl1 transcription) on all haematopoietic cell types with the highest expression observed on bone marrow progenitors (LSK cells; green) consistent with previous data [30] , then CLPs (orange), while pre-pro NK cells (Lin − c-kit − sca-1 + flt3 − IL-7Rα + ; red) and conventional NK cells (blue) expressed slightly lower levels ( Fig. 1c ). In the periphery, Mcl1 expression was found to increase as NK cells matured with M2 NK cells (red) expressing clearly higher levels of Mcl1 compared with M1 (blue) and Imm. (green) NK cells in the spleen ( Fig. 1d ) and liver ( Fig. 1e ), consistent with our mRNA data ( Fig. 1b ). We also verified Mcl1 expression in the TCR-β − NK1.1 + CD49b − hepatic resident NK cells (orange; Fig. 1e ) since their developmental origins and transcription factor requirements are distinct from conventional NK cells [31] . TCR-β − NK1.1 + CD49b − hepatic resident NK cells expressed an Mcl1 level equivalent to that of hepatic resident M1 NK cells ( Fig. 1e ). 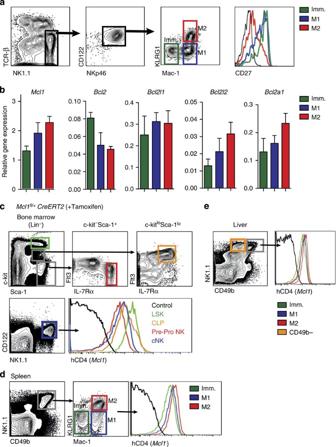Figure 1:Mcl1is expressed throughout NK cell development. (a) Peripheral NK cell subsets were sorted by flow cytometry from the spleen based on TCR-β, NK1.1, CD122, NKp46, CD27, Mac-1 and KLRG1 expression (Imm.—green; M1—blue; M2—red) and (b) expression ofMcl1,Bcl2,Bcl-x(Bcl2l1),Bcl-w(Bcl2l2) andA1(Bcl2a1) mRNA was determined by qPCR and normalized to HPRT. Data represent the mean±s.d. of two independent experiments. (c) Twelve-week-oldMcl1fl(loxp-hCD4)/+CreERT2mice were treated with tamoxifen by oral gavage and Mcl-1 expression (reflected by surface hCD4) analysed at 15 weeks by FACS in LSK cells (green), CLPs (orange), pre-pro NK cells (red) and conventional NK cells (blue) in the bone marrow. (d) Imm., M1 and M2 splenic NK cell subsets fromMcl1fl(loxp-hCD4)/+CreERT2mice were analysed forMcl1(hCD4) expression by FACS. Black histograms inc,drepresent mononuclear cells from tamoxifen-treatedMcl1+/+CreERT2mice.Mcl-1fl(loxp-hCD4)/+CreERT2mice were treated with tamoxifen by oral gavage. (d) Imm., M1 and M2 splenic NK cell subsets fromMcl1fl(loxp-hCD4)/+CreERT2mice were analysed forMcl1(hCD4) expression by FACS.Mcl-1fl(loxp-hCD4)/+CreERT2mice were treated with tamoxifen by oral gavage and (e) Imm. (green), M1 (blue) and M2 (red) and CD49b−(orange) hepatic NK cell subsets were analysed for Mcl-1 (hCD4) expression by FACS. Black histograms inc–frepresent mononuclear cells from tamoxifen-treatedMcl1+/+CreERT2mice. Data are representative of two independent experiments. Figure 1: Mcl1 is expressed throughout NK cell development. ( a ) Peripheral NK cell subsets were sorted by flow cytometry from the spleen based on TCR-β, NK1.1, CD122, NKp46, CD27, Mac-1 and KLRG1 expression (Imm.—green; M1—blue; M2—red) and ( b ) expression of Mcl1 , Bcl2 , Bcl-x ( Bcl2l1 ), Bcl-w ( Bcl2l2 ) and A1 ( Bcl2a1 ) mRNA was determined by qPCR and normalized to HPRT. Data represent the mean±s.d. of two independent experiments. ( c ) Twelve-week-old Mcl1 fl(loxp-hCD4)/+ CreERT2 mice were treated with tamoxifen by oral gavage and Mcl-1 expression (reflected by surface hCD4) analysed at 15 weeks by FACS in LSK cells (green), CLPs (orange), pre-pro NK cells (red) and conventional NK cells (blue) in the bone marrow. ( d ) Imm., M1 and M2 splenic NK cell subsets from Mcl1 fl(loxp-hCD4)/+ CreERT2 mice were analysed for Mcl1 (hCD4) expression by FACS. Black histograms in c , d represent mononuclear cells from tamoxifen-treated Mcl1 +/+ CreERT2 mice. Mcl-1 fl(loxp-hCD4)/+ CreERT2 mice were treated with tamoxifen by oral gavage. ( d ) Imm., M1 and M2 splenic NK cell subsets from Mcl1 fl(loxp-hCD4)/+ CreERT2 mice were analysed for Mcl1 (hCD4) expression by FACS. Mcl-1 fl(loxp-hCD4)/+ CreERT2 mice were treated with tamoxifen by oral gavage and ( e ) Imm. (green), M1 (blue) and M2 (red) and CD49b − (orange) hepatic NK cell subsets were analysed for Mcl-1 (hCD4) expression by FACS. Black histograms in c – f represent mononuclear cells from tamoxifen-treated Mcl1 +/+ CreERT2 mice. Data are representative of two independent experiments. Full size image Mcl1 is induced by γ C cytokines in a dose-dependent manner We next wanted to generate a model where Mcl1 was deleted specifically in NK cells via Cre-mediated deletion. The Ncr1 gene (encoding NKp46) is highly expressed in NK cells in all organs and, importantly, Ncr1 is not expressed to any significant level on other major immune cells. We investigated Mcl1 expression specifically in NK cells by crossing the Mcl1 fl-hCD4/+ mice with the Ncr1-iCre ( Ncr1-Cre ) mice [32] . The strict requirement for IL-15 on NK cell development in vivo prompted us to investigate the relationship between IL-15 and Mcl1 regulation in these cells. Culturing NK cells (TCR-β − NK1.1 + NKp46 + ) from Mcl1 fl-hCD4/+ Ncr1-Cre mice in graded concentrations of IL-15 resulted in a robust dose-dependent increase in Mcl1 (hCD4) expression ( Fig. 2a ). Western blot analysis of NK cell lysates confirmed that Mcl-1 and, to a lesser extent, Bcl-xL, but not Bcl-2, were elevated following IL-15 stimulation in vitro ( Fig. 2b ) and that these same proteins were degraded when IL-15 was withdrawn from NK cells that had been cultivated in a high concentration of IL-15 for 1 week ( Fig. 2c ). Since Bcl-xL was also increased in NK cells following IL-15 stimulation ( Fig. 2b ), we next determined the contribution of Bcl-xL to NK cell development in vivo by conditional deletion of Bcl-x (BCL2L1) in NK cells using the Bcl-x-loxP strain [33] . Bcl-x fl/fl Ncr1-Cre mice presented a normal proportion and number of NK cells in all organs examined indicating that Bcl-xL is not required for NK cell development in vivo ( Fig. 2d ). 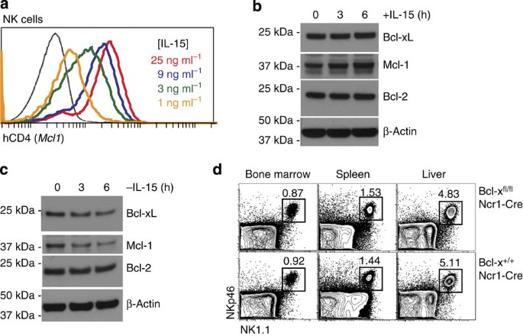Figure 2:Mcl1is induced by IL-15 in a dose-dependent manner. (a) Freshly isolated splenic NK cells (NKp46+NK1.1+TCR-β−) fromMcl1fl-hCD4/+Ncr1-Cremice were cultured for 18 h in the indicated concentrations of IL-15 and hCD4 (Mcl1) expression analysed by flow cytometry. (b) Splenic NK cells were sorted and stimulated for 0, 3 or 6 h with 40 ng ml−1IL-15. NK cell lysates were analysed for Bcl-xL, Mcl-1, Bcl-2 and β-actin (loading control) by western blotting. (c) Splenic NK cells were sorted and grown in 40 ng ml−1IL-15 for 7 days and then starved in media alone for 0, 3 or 6 h. NK cell lysates were analysed for Bcl-xL, Mcl-1, Bcl-2 and β-actin (loading control) by western blotting. (d) NK1.1+NKp46+cells inBcl-x+/+Ncr1-Creand Bcl-xfl/flNcr1-Cremice were analysed among TCR-β−mononuclear cells from the bone marrow, spleen and liver. Data are representative of four mice. Figure 2: Mcl1 is induced by IL-15 in a dose-dependent manner. ( a ) Freshly isolated splenic NK cells (NKp46 + NK1.1 + TCR-β − ) from Mcl1 fl-hCD4/+ Ncr1-Cre mice were cultured for 18 h in the indicated concentrations of IL-15 and hCD4 ( Mcl1 ) expression analysed by flow cytometry. ( b ) Splenic NK cells were sorted and stimulated for 0, 3 or 6 h with 40 ng ml −1 IL-15. NK cell lysates were analysed for Bcl-xL, Mcl-1, Bcl-2 and β-actin (loading control) by western blotting. ( c ) Splenic NK cells were sorted and grown in 40 ng ml −1 IL-15 for 7 days and then starved in media alone for 0, 3 or 6 h. NK cell lysates were analysed for Bcl-xL, Mcl-1, Bcl-2 and β-actin (loading control) by western blotting. ( d ) NK1.1 + NKp46 + cells in Bcl-x +/+ Ncr1-Cre and B cl-x fl/fl Ncr1-Cre mice were analysed among TCR-β − mononuclear cells from the bone marrow, spleen and liver. Data are representative of four mice. Full size image Mcl1 is essential for the generation of NK cells in mice Given the abundant expression of Mcl-1 driven by IL-15 in NK cells, we examined the importance of this pathway in vivo by deleting both Mcl1 alleles specifically in NKp46 + cells using the Ncr1-Cre mice. The result was striking; Mcl-1 fl/fl Ncr1-Cre + mice contained essentially no NK cells (TCR-β − NKp46 + NK1.1 + or TCR-β − CD49b + NK1.1 + ) in all organs examined ( Fig. 3a,b ). The few NK cells that remained in Mcl1 fl/fl Ncr1-Cre mice were Imm. ( Fig. 3c ). The Imm. stage of NK cell differentiation is the stage at which Ncr1-mediated Cre expression begins [32] and hence Mcl1 gene deletion is initiated ( Supplementary Fig. 2 ); thus, the appearance of only a very minor population of Imm. NK cells in Mcl-1 fl/fl Ncr1-Cre + mice confirms that the absence of Mcl-1 is incompatible with NK cell viability. 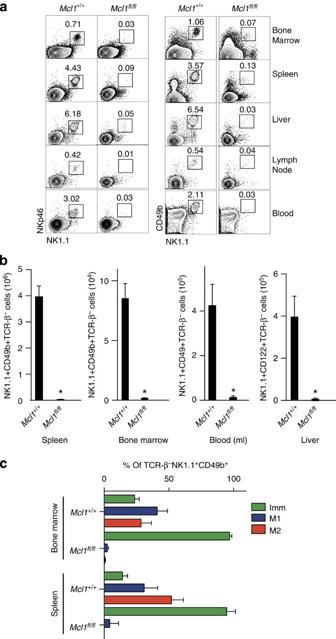Figure 3: Mcl-1 is essential for the generation of NK cellsin vivo. TheMcl1gene was specifically deleted in (NKp46+) cells by intercrossing theMcl1flandNcr1-Crestrains. (a) NK1.1+NKp46+and NK1.1+CD49b+cells inMcl1+/+Ncr1-CreandMcl1fl/flNcr1-Cremice were analysed among TCR-β−cells from the bone marrow, spleen, liver, lymph node and blood. Data in are representative of six mice. (b) TCR-β−NK1.1+CD49b+NK cells from the indicated organs were enumerated using the Advia blood analyser. Data are mean±s.e.m. of six mice of each genotype. Studentt-test;P>0.001. (c) Splenic TCR-β−NK1.1+CD49b+NK cells fromawere further analysed for Mac-1 and KLRG1 expression by flow cytometry and proportions of NK cell subsets (Imm.—green; M1—blue; M2—red) among these cells shown. Data incare mean±s.e.m. of six mice of each genotype. Figure 3: Mcl-1 is essential for the generation of NK cells in vivo . The Mcl1 gene was specifically deleted in (NKp46 + ) cells by intercrossing the Mcl1 fl and Ncr1-Cre strains. ( a ) NK1.1 + NKp46 + and NK1.1 + CD49b + cells in Mcl1 +/+ Ncr1-Cre and Mcl1 fl/fl Ncr1-Cre mice were analysed among TCR-β − cells from the bone marrow, spleen, liver, lymph node and blood. Data in are representative of six mice. ( b ) TCR-β − NK1.1 + CD49b + NK cells from the indicated organs were enumerated using the Advia blood analyser. Data are mean±s.e.m. of six mice of each genotype. Student t -test; P >0.001. ( c ) Splenic TCR-β − NK1.1 + CD49b + NK cells from a were further analysed for Mac-1 and KLRG1 expression by flow cytometry and proportions of NK cell subsets (Imm.—green; M1—blue; M2—red) among these cells shown. Data in c are mean±s.e.m. of six mice of each genotype. Full size image Outer mitochondrial membrane Mcl-1 inhibits NK cell death Mcl-1 has been recently proposed to contribute to cellular biogenesis in the inner mitochondrial membrane in addition to its known anti-apoptotic role in the outer membrane [24] . We next examined the ability of Mcl-1 (able to access the outer mitochondrial membrane and the mitochondrial matrix) and an Mcl-1 variant, Mcl-1 OM (expression restricted to the outer mitochondrial membrane) [24] in rescuing NK cell survival in the absence of wild-type Mcl-1. To do this, Mcl-1 fl/fl Ncr1-Cre LSK cells were transduced in vitro with retrovirus encoding vector alone, Mcl-1 or Mcl-1 OM and all co-expressing green-fluorescent protein; GFP; Fig. 4a ). Total LSK cells were then cultured for 21 days in 50 ng ml −1 IL-15 and analysed for NK cell generation. Despite similar transduction efficiency to Mcl-1, Mcl-1 fl/fl Ncr1-Cre LSKs transduced with vector alone (GFP) failed to generate NK cells, underlining the requirement of Mcl-1 for NK cell genesis, even in high concentrations of IL-15. In contrast, ectopic expression of either Mcl-1 or Mcl-1 OM was equally efficient in rescuing NK cell development from Mcl-1 fl/fl Ncr1-Cre LSK cells in vitro ( Fig. 4a ). NK cell development under these conditions was robust and independent of Mcl-1 expression in the mitochondrial matrix suggesting the primary defect following loss of Mcl-1 in NK cells is the inability to antagonize the pro-apoptotic BH3-only and BAX/BAK proteins and not in mitochondrial fusion or cellular biogenesis. Collectively, these results clearly indicate that Mcl-1 is the principle antagonist of apoptosis in NK cells and are consistent with our in vitro observation that Mcl-1 levels are proportional to NK cell viability following IL-15 withdrawal ( Fig. 2c ) [14] . 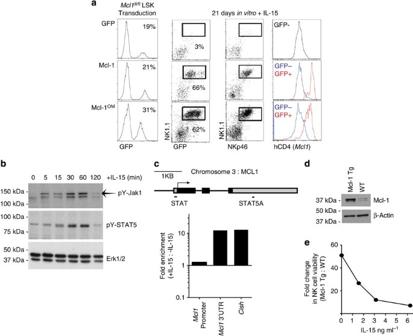Figure 4: Outer mitochondrial membrane Mcl-1 protects from apoptosis. (a) LSK cells were sorted by flow cytometry from the bone marrow ofMcl1fl/flNcr1-Cremice and transduced using retrovirus encoding Mcl-1, Mcl-1OM(outer mitochondrial membrane only) or empty vector (GFP). Total lin−sca-1−c-kit−(LSK cells) were analysed for transduction efficiency (GFP) by flow cytometry and then cultured for 21 days in 50 ng ml−1IL-15. Cultures were then analysed for GFP and hCD4 expression among resulting NK cells. Data are representative of two experiments. (b) Splenic NK cells were sorted and grown in 40 ng ml−1IL-15 for 7 days and then starved in media alone for 5 h. NK cells were then stimulated with 40 ng ml−1IL-15 for the indicated time. NK cells were then lysed and analysed for tyrosine-phosphorylated Jak1, STAT5 and total ERK1/2 (loading control) by western blotting. Blots are representative of five independent experiments. (c) STAT5 ChIP. A diagram of STAT-binding sites in theMcl1locus is shown. Splenic NK cells were sorted and grown in 40 ng ml−1IL-15 for 7 days and then starved in media alone or maintained in 40 ng ml−1IL-15 for 5 h. STAT5 ChIP was preformed on formaldehyde-fixed NK cell lysates. Data represent fold enrichment ofMcl1promoter or 3′-UTR DNA sequences in IL-15 treated versus starved NK cell lysates. Enrichment ofCishis used as a positive control. Histograms are representative of two independent experiments. (d) Splenic NK cells from Vav-Mcl-1 transgenic and wild-type (WT) mice were sorted and grown in 40 ng ml−1IL-15 for 7 days. NK cell lysates were analysed for Mcl-1 and β-actin (loading control) by western blotting. (e) Vav-Mcl-1 transgenic mice (Mcl-1 Tg) and WT NK cells were cultured for 48 h in the indicated doses of IL-15. Data represent fold difference in NK cell viability (PI−) comparing Vav-Mcl-1 transgenic mice to wild type. Figure 4: Outer mitochondrial membrane Mcl-1 protects from apoptosis. ( a ) LSK cells were sorted by flow cytometry from the bone marrow of Mcl1 fl/fl Ncr1-Cre mice and transduced using retrovirus encoding Mcl-1, Mcl-1 OM (outer mitochondrial membrane only) or empty vector (GFP). Total lin − sca-1 − c-kit − (LSK cells) were analysed for transduction efficiency (GFP) by flow cytometry and then cultured for 21 days in 50 ng ml −1 IL-15. Cultures were then analysed for GFP and hCD4 expression among resulting NK cells. Data are representative of two experiments. ( b ) Splenic NK cells were sorted and grown in 40 ng ml −1 IL-15 for 7 days and then starved in media alone for 5 h. NK cells were then stimulated with 40 ng ml −1 IL-15 for the indicated time. NK cells were then lysed and analysed for tyrosine-phosphorylated Jak1, STAT5 and total ERK1/2 (loading control) by western blotting. Blots are representative of five independent experiments. ( c ) STAT5 ChIP. A diagram of STAT-binding sites in the Mcl1 locus is shown. Splenic NK cells were sorted and grown in 40 ng ml −1 IL-15 for 7 days and then starved in media alone or maintained in 40 ng ml −1 IL-15 for 5 h. STAT5 ChIP was preformed on formaldehyde-fixed NK cell lysates. Data represent fold enrichment of Mcl1 promoter or 3′-UTR DNA sequences in IL-15 treated versus starved NK cell lysates. Enrichment of Cish is used as a positive control. Histograms are representative of two independent experiments. ( d ) Splenic NK cells from Vav-Mcl-1 transgenic and wild-type (WT) mice were sorted and grown in 40 ng ml −1 IL-15 for 7 days. NK cell lysates were analysed for Mcl-1 and β-actin (loading control) by western blotting. ( e ) Vav-Mcl-1 transgenic mice (Mcl-1 Tg) and WT NK cells were cultured for 48 h in the indicated doses of IL-15. Data represent fold difference in NK cell viability (PI − ) comparing Vav-Mcl-1 transgenic mice to wild type. Full size image IL-15 directly regulates Mcl1 via STAT5 binding the 3′-UTR To understand how the dynamic regulation of Mcl1 in response to IL-15 is achieved, we next investigated the molecular pathways activated by IL-15 in NK cells. IL-15 stimulation of NK cells resulted in the rapid induction of Jak1 and STAT5A/B phosphorylation that peaked between 30 and 60 min ( Fig. 4b ). STAT5 is a transcription factor that dimerizes upon phosphorylation and translocates to the nucleus where it can drive the expression of a large number of genes via binding an evolutionarily conserved TTC(T/C)N(G/A)GAA motif [34] , [35] . We identified a conserved STAT motif in the promoter and a conserved STAT5 motif in 3′-UTR of Mcl1 ( Fig. 4c ). To determine whether STAT5 directly bound to Mcl1 in NK cells, we cultivated NK cells in a high concentration of IL-15 to induce STAT5 phosphorylation and performed chromatin immunoprecipitation (ChIP) using STAT5 antiserum. NK cells not stimulated with IL-15 were used as a negative control as these cells displayed negligible STAT5 phosphorylation with western blot. STAT5 ChIP confirmed a robust enrichment of the 3′-UTR sequence of Mcl1 but not the promoter in NK cells stimulated with IL-15 compared with untreated NK cells indicating that STAT5 directly binds the 3′-UTR of Mcl1 ( Fig. 4c ). Enrichment of the well-characterized STAT5 target gene Cish (cytokine-inducible SH2-containing protein) was used as a positive control as this gene has multiple TTC(T/C)N(G/A)GAA motifs in its promoter [36] ( Fig. 4c ). Given that IL-15 directly maintains NK cell viability by driving Mcl-1 expression via STAT5, we next determined whether the requirement for IL-15 could be overcome by transgenic expression of Mcl1 in NK cells. NK cells from Vav-Mcl-1 transgenic (Mcl-1 Tg) mice [37] displayed greatly enhanced Mcl-1 protein levels compared with littermate controls ( Fig. 4d ) and when cultured in limiting concentrations of IL-15 Mcl-1 Tg NK cell survival was 10- to 50-fold greater than control NK cells ( Fig. 4e ). Taken together, these data identify Mcl1 as a STAT5 target gene in NK cells and highlight the direct link between IL-15 signalling and NK cell survival. Absence of innate cytotoxicity in NK lymphopenic mice NK cells were the first ILCs described owing to their spontaneous ability to kill target cells that had altered expression of major histocompatibility complex (MHC)-I (non-self MHC-I or reduced/absent MHC-I) and this role has since been extended to the killing of cells expressing stress-induced activating ligands [38] , [39] . NK cells are also potent producers of pro-inflammatory cytokines, namely interferon (IFN)-γ upon pathogen encounter. Studying the in vivo role of NK cells has largely relied on NK cells being depleted with anti-NK1.1 antibody since a mouse strain specifically lacking NK cells was, until now, unavailable. We next examined some functional consequences of the complete loss of NK cells in Mcl1 fl/fl Ncr1-Cre mice. Following injection with B16F10 murine melanoma cells (lacking MHC-I but expressing DNAM-1 ligand, CD155), Mcl1 fl/fl Ncr1-Cre mice needed to be killed after 12 days because of acute onset of respiratory distress. Post-mortem analysis revealed that the lungs of these animals were overwhelmed with melanoma metastases, whereas metastases were rarely observed in similarly challenged control mice ( Mcl1 +/+ Ncr1-Cre ; Fig. 5a,b ). B16F10 is not thought to be a particularly metastatic variant of B16 and has been classically used to measure experimental lung metastasis; however, we discovered that at the low dose used, the tumour cells metastasized extensively and were located in additional sites in Mcl1 fl/fl Ncr1-Cre mice. This included the liver, bone marrow, kidney and lymph nodes, whereas metastases at these sites were never observed in control mice ( Fig. 5c,d ). 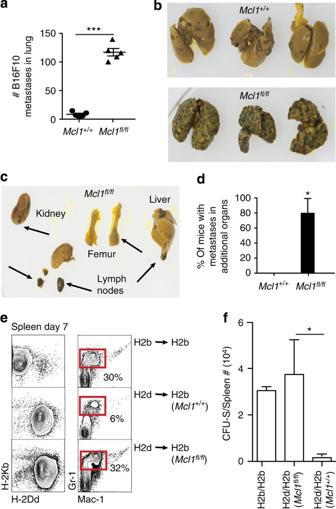Figure 5: Absence of innate cytotoxicity in NK lymphopenic mice. Mcl1+/+Ncr1-Cre(negative control) andMcl1fl/flNcr1-Cremice were injected i.v. with 40,000 B16F10 melanoma cells. On day 12, mice were killed and peripheral organs analysed for B16F10 metastases. (a) The frequency of lung metastases was enumerated. Data represent mean±s.e.m. of five mice of each genotype. Student’st-test; ***P<0.0001. (b) Representative whole mounts of lungs are shown. (c) Representative whole mounts of diseased bone marrow, liver, kidney and lymph nodes fromMcl1fl/flNcr1-Cremice are shown. (d) The frequency of mice with B16F10 metastases in additional organs was enumerated. (e) A total of 1.5 × 107allogeneic (H-2d) bone marrow cells were transplanted into lethally irradiatedMcl1fl/+Ncr1-CreandMcl1fl/flNcr1-Cre(H-2b) recipients and (e) splenic myeloid (Gr-1+) reconstitution analysed by flow cytometry. (f) CFU-S were enumerated after 8 days. A total of 1.5 × 107autologous (H-2b) bone marrow cells (H-2b) were transplanted into lethally irradiatedMcl1fl/+Ncr1-Cremice as a control. Data ineare representative and infare the mean±s.e.m. of three mice of each genotype. Student’st-test; *P<0.03. Figure 5: Absence of innate cytotoxicity in NK lymphopenic mice. Mcl1 +/+ Ncr1-Cre (negative control) and Mcl1 fl/fl Ncr1-Cre mice were injected i.v. with 40,000 B16F10 melanoma cells. On day 12, mice were killed and peripheral organs analysed for B16F10 metastases. ( a ) The frequency of lung metastases was enumerated. Data represent mean±s.e.m. of five mice of each genotype. Student’s t -test; *** P <0.0001. ( b ) Representative whole mounts of lungs are shown. ( c ) Representative whole mounts of diseased bone marrow, liver, kidney and lymph nodes from Mcl1 fl/fl Ncr1-Cre mice are shown. ( d ) The frequency of mice with B16F10 metastases in additional organs was enumerated. ( e ) A total of 1.5 × 10 7 allogeneic (H-2d) bone marrow cells were transplanted into lethally irradiated Mcl1 fl/+ Ncr1-Cre and Mcl1 fl/fl Ncr1-Cre (H-2b) recipients and ( e ) splenic myeloid (Gr-1 + ) reconstitution analysed by flow cytometry. ( f ) CFU-S were enumerated after 8 days. A total of 1.5 × 10 7 autologous (H-2b) bone marrow cells (H-2b) were transplanted into lethally irradiated Mcl1 fl/+ Ncr1-Cre mice as a control. Data in e are representative and in f are the mean±s.e.m. of three mice of each genotype. Student’s t -test; * P <0.03. Full size image Residual NK cell activity following whole-body γ-irradiation is associated with bone marrow allograft rejection [40] , [41] . Consistent with the previous finding, C57BL/6 (H-2b) recipient mice lacking NK cells ( Mcl1 fl/fl Ncr1-Cre ) possessed significantly more splenic monocytes and spleen colony-forming units (CFU-S) on day 8 post transplantation with allogeneic BALB/c (H-2d) bone marrow cells compared with NK cell-proficient control recipients ( Mcl1 +/+ Ncr1-Cre ; Fig. 5e,f ). CFU-S counts are a reflection of bone marrow engraftment and the fact that recipients lacking NK cells possessed similar CFU-S counts after allogeneic bone marrow transplantation as C57BL/6 mice receiving syngeneic bone marrow (H-2b) demonstrates that Mcl-1-dependent survival of NK cells is critical for the early clearance of MHC-mismatched bone marrow and a contributing factor in bone marrow transplant outcomes. NK lymphopenia protects mice from lethal sepsis Sepsis is a systemic inflammatory response to bacterial infection resulting in the death of over a million humans annually. Polymicrobial sepsis induced by cecal ligation and puncture (CLP) is the most common murine model of bacterial sepsis [42] . This model induces a hyperinflammatory response by innate immune cells, characterized by high levels of IL-6, tumour necrosis factor and MCP-1 typically resulting in death within 48 h (ref. 43 ). To investigate the contribution of NK cells in CLP-mediated sepsis, we compared mice with varying degrees of NK cell deficiency from including Mcl1 fl/fl Ncr1-Cre (~0% NK cells), anti-αasialoGM1-treated C57BL/6 (30–40% NK cells), anti-NK1.1-treated C57BL/6 (~10% in NK cells) and control C57BL/6 Mcl1 +/+ Ncr1-Cre (100% NK cells; Fig. 6a ). Strikingly, Mcl1 fl/fl Ncr1-Cre mice were resistant to toxic shock induced by CLP compared with control mice, similarly mice depleted of NK cells by antibody treatment (anti-NK1.1 and anti-αasialoGM1; Fig. 6a ) were also largely protected ( Fig. 6b ). The presence or absence of NK cells had no bearing on the bacterial load with no differences in bacteria colony forming units observed in the blood at this early time point ( Fig. 6c ). The protection offered by the absence of NK cells was characterized by a significant reduction in IFN-γ and IL-6 protein levels in the serum 12 h following CLP ( Fig. 6d,e ). This finding indicates that an NK cell-dependent pro-inflammatory cytokine response contributes to the lethality following CLP in mice and that even a 50% reduction in NK cells is effective in reducing the incidence of death due to septic shock. 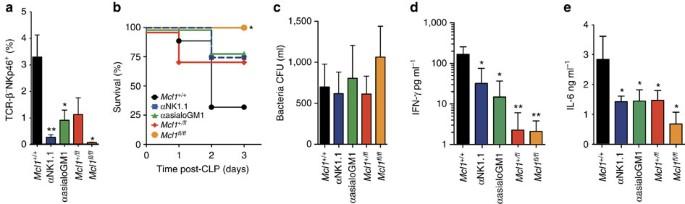Figure 6: NK lymphopenia protects mice from lethal sepsis. CLP was performed on mice lacking NK cells (Mcl1fl/flNcr1-Cre) or with reduced numbers of NK cells (anti-NK1.1 or anti-αasialoGM1 antibody treated). (a) NK cell frequencies were enumerated in the blood of the indicated mice on the day of CLP. Student’st-tests using the Sidak–Bonferroni method; **P<0.01; *P<0.03. (b) Kaplan–Meier survival curve following CLP-induced septic shock. Mantel–Cox test; *P<0.04. (c) Bacteria CFUs from peripheral blood were enumerated on agar plates 12 h after CLP induction. (d) Serum IFN-γ and (e) IL-6 levels were measured at 12 h after CLP.t-tests using the Sidak–Bonferroni method; **P<0.009; *P<0.05. Data are mean±s.e.m. of five to six mice of each genotype per treatment group. Figure 6: NK lymphopenia protects mice from lethal sepsis. CLP was performed on mice lacking NK cells ( Mcl1 fl/fl Ncr1-Cre ) or with reduced numbers of NK cells (anti-NK1.1 or anti-αasialoGM1 antibody treated). ( a ) NK cell frequencies were enumerated in the blood of the indicated mice on the day of CLP. Student’s t -tests using the Sidak–Bonferroni method; ** P <0.01; * P <0.03. ( b ) Kaplan–Meier survival curve following CLP-induced septic shock. Mantel–Cox test; * P <0.04. ( c ) Bacteria CFUs from peripheral blood were enumerated on agar plates 12 h after CLP induction. ( d ) Serum IFN-γ and ( e ) IL-6 levels were measured at 12 h after CLP. t -tests using the Sidak–Bonferroni method; ** P <0.009; * P <0.05. Data are mean±s.e.m. of five to six mice of each genotype per treatment group. Full size image NK cells evolved before adaptive lymphocytes and lack the somatically rearranged antigen receptors that control the development and survival of B and T cells [44] , [45] . Here we demonstrate conclusively that NK cells instead rely on a non-redundant pathway for IL-15 in directly regulating the expression of the anti-apoptotic protein Mcl-1 via STAT5 binding to the 3′ UTR for their viability in vivo . Mcl-1 expression in NK cells requires IL-15 and is tightly regulated suggesting that changes in the levels of these cytokines will greatly impact on NK cell homeostasis in vivo . IL-15 is derived from both parenchymal and hematopoietic cells and plays an integral role in the homeostasis of various T-cell subsets such as γ/δ T cells, NKT cells, CD8αα T cells as well as innate lymphocytes [46] , [47] . A similar mechanism of IL-15-dependent Mcl-1 regulation in these cell types is also likely. Other members of the Bcl-2 family have been shown to be upregulated in lymphocytes following stimulation with IL-15 and proposed to antagonize the pro-apoptotic BH3-only and BAX/BAK proteins to prevent cell death [48] , [49] . Our observation and those of others indicate that Bcl-2 family members in addition to Mcl-1 are upregulated in NK cells by cytokines that stimulate γ C chain containing receptors; however, these apoptosis inhibitors must function in synergy with Mcl-1 to promote NK cell survival [14] , [22] . For example, while we found Bcl-xL to be completely redundant in maintaining steady-state NK cell survival, this is not to say that induction of Bcl-xL in NK cells is irrelevant for NK cell survival during different circumstances such as inflammation. It is interesting that the requirement for Mcl-1 in NK cell survival appears greater than that of STAT5, a major transcriptional activator downstream of IL-15 signalling that we found to bind the 3′-UTR of Mcl1 . In vivo deletion of STAT5 specifically in NK cells via the Ncr1-Cre transgene (using a bacterial artificial chromosome approach) only resulted in three to sixfold reduction in peripheral NK cell numbers in vivo [50] , which is consistent with earlier germ-line deletion studies [51] and an order of magnitude less than the reduction in NK cells observed in Mcl1 fl/fl Ncr1-Cre mice (up to 100-fold reduction in some organs). This suggests that STAT3, which is phosphorylated following IL-15 stimulation in NK cells, may also contribute to Mcl-1 expression in the absence of STAT5, as a similar pathway is proposed to exist in various tumour cells [52] , [53] . STAT3 phosphorylation is also induced following stimulation of IL-21R/γ C heterodimers [54] thus it will be interesting to investigate if the synergy between IL-15 and IL-21 converge at the level of STAT3 activation leading to Mcl1 expression. We are only now beginning to understand the intrinsic pathways required for NK cell homeostasis. Following upregulation of Id2 in pre-pro NK cells [7] , expression of the IL-2/15Rβ (CD122) is acquired and NK cells become dependent on IL-15. The near total loss of NK cells following Mcl1 deletion may suggest that their dependency on Mcl-1 for survival is more stringent than that of B and T cells, since specific deletion of Mcl1 using CD19-Cre (B-cell-specific) and Lck-Cre (T-cell-specific) resulted in a less dramatic loss of these cell types in vivo [22] than what we observed for NK cells. It remains possible that this may also reflect the efficiency of Cre expression from the respective transgenes. The aforementioned conclusion would, however, explain why transgenic Bcl-2 overexpression failed to rescue NK cell development in γ C −/− mice but could (partially) rescue T-cell development in these animals [55] . Furthermore, specific deletion of STAT5 in lymphoid progenitors via Rag1-Cre expression results in an absence of Pro-B cells that can also be rescued by Bcl-2 overexpression [56] . In these ‘rescued’ STAT5-null Pro-B cells, Mcl-1 protein was absent compared with STAT5-sufficient Pro-B cells suggesting a role for STAT5 in directly inducing Mcl-1 in the B lineage in response to IL-7 (ref. 56 ). The fidelity and efficiency of Cre-expression in the Ncr1-iCre strain is paramount to our success in generating an NK cell null mouse model. This clear and sustained lack of innate effector functions in Mcl1 fl/fl Ncr1-Cre mice offers the most relevant model to date in addressing the contribution of NK cells in mammalian immune defense. This model does not require in vivo administration of antibodies or diphtheria toxin to deplete NK cells or affect additional cell types, caveats of all current approaches [4] , [5] , [6] , [57] , [58] , [59] . Functionally, our results demonstrate that NK cells are a rapid source of pro-inflammatory cytokines following detection of bacteria in vivo contributing to septic shock and are central to the clearance of cells lacking self-MHC-I expression in vivo. Collectively, these findings unequivocally demonstrate for the first time that induction of anti-apoptotic Mcl-1 expression by IL-15 is required for the survival of NK cells in vivo . Mice Mcl1-loxp-hCD4 (refs 25 , 26 ), Rosa26-CreERT2 (TaconicArtemis), Bcl-x-loxp [33] Rosa26-(loxP-stop-loxP)yfp [60] Vav-Mcl1 Tg [37] and Ncr1-iCre mice [32] were bred and maintained at the Walter and Eliza Hall of Medical Research. The Mcl-1-loxp-hCD4 , Rosa26-CreERT2, Vav-Mcl1 Tg and Rosa26-EYFP mice were generated on a C57BL/6 background using C57BL/6-derived ES cells. The Ncr1-iCre mice were generated on a mixed C57BL/6 × 129SV background using 129SV-derived ES cells and then backcrossed with C57BL/6 mice for at least eight generations. The relevant Animal Ethics and Experimentation Committees approved animal experiments according to the guidelines of the National Health and Medical Research Council Australia. Both female and male mice aged between 8 and 15 weeks of age were used in this study. Age and sex matching was performed for each independent experiment. Flow cytometry and cell sorting Antibodies specific for NK1.1 (PK136; 1:400), Sca-1 (E13-161.7; 1:200), c-kit (2B8; 1:500), hCD4 (RPAT4; 1:100), Gr-1 (RB6-8C5; 1:500), CD244.2 (244F4; 1:200), CD19 (1D3; 1:500), CD3 (KT31.1; 1:500), CD122 (TM-β1; 1:200), NKp46 (29A1.4; 1:100), Flt3 (A2F10.1; 1:100), CD127 (A7R34; 1:200), CD11b (M1/70; 1:800), TCR-β (H57-5921; 1:500), CD45.2 (104; 1:500, KLRG1 (2F1; 1:100), CD27 (LG.7F9; 1:200), H-2b (AF6-88.5.3.3; eBioscience; 1:100) H-2d (34-2-12; 1:100) and CD49b (DX5; 1:200 and HMa2; 1:200) were from BD PharMingen unless stated otherwise. Single-cell suspensions were prepared by forcing of organs through 70-μM sieves. Lymphocytes from the liver were isolated by suspension in isotonic percoll (Amersham Pharmacia Biotech) and centrifugation at 1,800 g . For flow cytometry, single-cell suspensions were stained with the appropriate monoclonal antibody in phosphate-buffered saline (PBS) containing 2% (vol/vol) fetal calf serum (FCS). FACS Verse, Fortessa and AriaII (BD Biosciences) were used for cell sorting and analysis, with dead cells excluded by propidium iodide staining. Depletion of differentiated cells was performed by incubating bone marrow suspensions with a cocktail of rat monoclonal antibody against CD3 (KT3), CD8 (53-6.7), CD19 (1D3), Ter119 (TER119), CD11b (M1/70) and Ly6G (1A8). Supernatants from these hybridoma cultures were generated in house, titrated on bone marrow suspensions and visualized with anti-rat FITC or anti-rat Al700 to control for any variability in labelling efficiency over time. Antibodies were added to the cocktail at the dilution found to give optimal labelling by FACS, constituting 2–10% of the final cocktail volume. The bone marrow suspension was then incubated with polyclonal sheep anti-rat IgG magnetic beads at a ratio of eight beads per cell, and bead-bound cells magnetically depleted. Remaining differentiated cells were visualized by staining with anti-rat Al700. All single-cell suspensions were diluted in PBS before analysis and enumeration using the Advia hematology analyzer (Siemens). In vivo analysis of NK cells Melanoma metastasis: 4 × 10 4 B16F10 melanoma cells (perforin-sensitive, FasL- and TRAIL-insensitive, H-2 b ; ATCC) were injected i.v. into mice and monitored for respiratory difficulty and weight loss. At 12 days, mice were killed. Lymphoid organs, kidney, liver and lungs were harvested, fixed in Bouin’s solution and B16F10 metastases counted [61] . Allogeneic bone marrow transplants: 1.5 × 10 7 allogeneic (H-2d) and syngeneic (H-2b) total bone marrow cells were injected i.v. into lethally irradiated mice (2 × 5.5 Gy). Eight days later, mice were killed, and lymphoid organs harvested and analysed for H-2d haematopoietic engraftment. Colony assays (CFU-S) were performed with 0.6% agar and 2 × DME+40% FCS. In all, 1 × 10 5 splenocytes per plate were added into a tube containing equal concentrations of 2 × DME/FCS and Difco Bacto Agar. In all, 100 μl of GM-CSF made up at 100 ng ml −1 was added to the plate. Plates were incubated at 10% CO 2 for 7 days and colonies were counted using a light microscope. Colonies were classified as greater than 50 cells [62] , [63] . CLP was performed at QIMR Berghofer Medical Research Institute. Briefly, mice were anesthetized with isoflurane, the abdomen was shaved, disinfected using betadine antiseptic spray and a midline incision made. The cecum was externalized with a cotton bud and 75% was ligated and punctured once using a 25-gauge needle to extrude a small amount of cecal content. The cecum was returned to the abdomen, the peritoneal was closed via continuous suture and the skin was sealed using an auto clip wound clip applier (Becton Dickinson). Buprenorphin (Reckitt Benckiser Pharmaceutical) was applied at 0.05 mg per kg body weight at the incision site for postoperative analgesia [64] . NK cell depletion was performed by treating mice with 100 μg of purified antibody with anti-NK1.1 (PK136) or anti-αasialoGM1 antibody (Wako Pure Chemical Industries) at day −3 and day 0 before CLP. Tamoxifen oral gavage was performed as in refs 25 , 26 . In vitro NK cell assays NK cell cultivation was performed in Iscove’s modified Dulbecco’s medium supplemented with 10% (vol/vol) FCS plus gentamycin (50 ng ml −1 ; Sigma) and 40 ng ml −1 recombinant hIL-15 (Peprotech). NK cells cocultured (1 × 10 5 of each) in vitro with various doses of hIL-15 (Peprotech) for 5 days. Mcl-1 induction studies were performed by culturing purified Mcl1 fl-hCD4/+ Ncr1-Cre NK cells in hIL-15 (Peprotech) in 96-well, flat-bottomed plates. Live and dead cells were discriminated by staining with propidium iodide. Bone marrow LSK cell transduction was performed using retrovirus packaged in 293T cells. Briefly, 10-cm tissue culture plates containing 80% confluent 293T cells were treated with chloroquine (25 mM) for 30 min at 37 °C before transfection with plasmids encoding eco-MLV (0.2 μg ml −1 ), gag-pol (0.3 μg ml −1 ) and either GFP, Mcl-1 or Mcl-1 OM (ref. 14 ) (1 μg ml −1 ) using CaCl 2 (20 mM) and HBSS (2 × ) [24] . LSKs were transduced with a combination of RetroNectin (Takara) and spin inoculation. Twelve well non-tissue culture plates were coated for 12 h with RetroNectin (4 mg cm −2 in PBS) at 4 °C before blocking with PBS containing 2% (wt/vol) bovine serum albumin (BSA) at 25 °C. Viral supernatant (2 ml) was added and plates were then centrifuged for 2 h at 37 °C and 1,200 g . LSKs were cultured for 48 h in IL-15 (50 ng ml −1 ) at 2 × 10 6 cells per ml. Polybrene (2.5 μg ml −1 ) was added to these cultures, and the cultures added to each virus coated well from above after the viral supernatant was removed. Cells were then cultured for 12 h at 37 °C. Fresh wells were then coated with 2 ml viral supernatant as above, and the LSK cultures transferred to these wells for 12 h at 37 °C. Cultures were transferred to tissue culture-treated plates after this second round of transduction, and infection efficiency was determined using flow cytometry of GFP expression. Quantitative PCR and STAT5 ChIP Total RNA from 3 × 10 5 Imm. M1 and M2 NK cells were purified using RNeasy mini columns (Qiagen). SuperScript II reverse transcriptase (Roche) was used for first-strand cDNA synthesis according to the manufacturer’s instructions. Quantitative PCR was performed using Sensimix SYBR HI-ROX (Bioline) and the Bio Rad CFX384 detection system and software (Bio Rad). Primers used ( Mcl1 , Bcl2 , Bcl-x ( Bcl2l1 ), Bcl-w ( Bcl2l2 ) and A1 ( Bcla1 ), Puma (Bbc3), Noxa (Pmaip1), Bim (Bcl211)) have been described [65] . The relative expression of each gene was normalized to Hprt . For STAT5 ChIP, 1.5 × 10 7 in vitro expanded splenic NK cells were cultured in IL-15 (40 ng ml −1 ) or media alone for 5 h. NK cells were then crosslinked for 10 min in presence of 1% paraformaldehyde (Sigma) in PBS then lysed (1% SDS+1 mM EDTA+proteases inhibitors). Crosslinked DNA was sonicated with the Branson sonifier 250 (Branson). Lysates were incubated overnight with 10 μg of Pan human/mouse Stat5a/b antibody (R&D). In all, 100 μl of Protein G Dynabeads (Invitrogen) were added and incubated for 2 h at 4 °C under gentle rotation. Unbound chromatin was removed using a series of five washes (low salt, high salt, liCL and 2xTE). Following elution, bound chromatin was reverse cross-linked and subjected to phenol/chloroform immunoprecipitation. Recovered DNA was resuspended in TE buffer and enrichment for specific region of the genome was measured with real-time PCR using the primers described ( Supplementary Table 1 ). Raw C t values are shown in Supplementary Table 2 . Immunoblotting Protein extracts were prepared in RIPA buffer (300 mM NaCl, 2% IGEPAL CA-630, 1% deoxycholic acid, 0.2% SDS, 100 mM Tris–Hcl pH 8.0) and 30 μg of protein was loaded into NuPAGE 10% Bis-Tris gels. Western blotting was performed according to the standard procedures. Blots were probed with the following antibodies: Mcl-1 (1:1,000 clone 19C4-15, WEHI mAb lab); Bcl-2 ((1:500) clone 7, BD Biosciences); Bcl-xL ((1:1,000) polyclonal, BD Biosciences); pY-STAT5 (Tyr694; 1:1,000 Millipore), pY-Jak1 (1:1,000 1022/1023; Invitrogen), Erk1/2 (1:1,000 Cell Signaling), Bim (1:2,000 polyclonal, Enzo Life Sciences); and β-actin (1:2,000 clone AC-74, Sigma). Uncropped Immunoblots are displayed in Supplementary Fig. 3 . Statistical analysis A standard Student’s t -test with two-tailed distributions for two samples with equal variance was used for statistical analysis. P values are provided. In Fig. 6b significance of survival differences were determined using Mantel–Cox test, whereas for Fig. 6c,e,f , t -tests using the Sidak–Bonferroni method were performed. How to cite this article: Sathe, P. et al. Innate immunodeficiency following genetic ablation of Mcl1 in natural killer cells. Nat. Commun. 5:4539 doi: 10.1038/ncomms5539 (2014).